Pandemic 2009 H1N1 vaccine protects against 1918 Spanish influenza virus The 1918 influenza A virus caused the most devastating pandemic, killing approximately 50 million people worldwide. Immunization with 1918-like and classical swine H1N1 virus vaccines results in cross-protective antibodies against the 2009 H1N1 pandemic influenza, indicating antigenic similarities among these viruses. In this study, we demonstrate that vaccination with the 2009 pandemic H1N1 vaccine elicits 1918 virus cross-protective antibodies in mice and humans, and that vaccination or passive transfer of human-positive sera reduced morbidity and conferred full protection from lethal challenge with the 1918 virus in mice. The spread of the 2009 H1N1 influenza virus in the population worldwide, in addition to the large number of individuals already vaccinated, suggests that a large proportion of the population now have cross-protective antibodies against the 1918 virus, greatly alleviating concerns and fears regarding the accidental exposure/release of the 1918 virus from the laboratory and the use of the virus as a bioterrorist agent. The 1918 influenza A virus genome encompasses a constellation of genes that result in a highly pathogenic and lethal virus that is believed to be responsible for the most devastating pandemic of the twentieth century, resulting in an estimated 50 million deaths worldwide. The reconstruction and characterization of the formerly extinct 1918 virus have greatly enhanced our knowledge of virulence factors and pathogenesis determinants of this virus and other pandemic influenza viruses [1] , facilitating the rapid assessment of the potential virulence of the 2009 H1N1 pandemic virus [2] . Nevertheless, the same study raised some anxieties because of its potential for dual use [1] , [3] , that is, this virus could be used not only to understand how to prevent and treat severe influenza virus infections but also to construct potential bioterrorist agents. Questions were also raised about the possible consequences of an unwanted accidental release from the laboratory [3] . Although these concerns could be addressed by the use of biocontainment facilities and the availability of effective antivirals, currently no licensed vaccine exists against the 1918 pandemic influenza virus. Inactivated and live attenuated vaccines are the main means of protection against influenza viruses in the general human population. There is extensive knowledge on vaccine safety, and vaccines are widely used every year to immunize against seasonal influenza strains. The emergence of the 2009 H1N1 pandemic influenza A virus and the potential devastating consequences of a more virulent second wave prompted governments to work together with vaccine manufacturers to rapidly develop a pandemic strain vaccine that has now become available worldwide. It is estimated that millions of individuals have now been vaccinated with this novel vaccine strain. As a consequence of continued global circulation of the new H1N1 virus, and as it remains the predominant circulating influenza A strain in the Northern and Southern Hemisphere [4] , [5] , the current recommendation from World Health Organization includes the pandemic strain as part of the 2010–2011 trivalent vaccine formulation [5] . Recent studies have demonstrated that 1918-like and classical swine H1N1 viruses share antigenic similarities [6] , [7] , [8] , [9] . Unexpectedly, the 1918 and 2009 H1N1 haemagglutinin (HA) proteins were found to have the highest homology in the known antigenic sites. In this paper, we demonstrate that immunization of mice and humans with the novel 2009 H1N1 vaccine strain results in the production of antibodies that crossreact with the 1918 virus, and that these antibodies are capable of conferring full protection in mice from a 1918 lethal challenge. Passive transfer of human 2009 H1N1-positive sera or mouse 2009 H1N1 HA-specific monoclonal antibodies (mAbs) was sufficient to protect mice from the lethality of 1918 virus infection. Our data indicate that vaccination or previous exposure to the 2009 H1N1 pandemic virus elicits cross-protective antibodies in the general human population, and that antigenic site Sa is an important cross-protective epitope between these two viruses. More important, our results should ease concerns of accidental release of the 1918 virus from the laboratory, or its use as a bioterrorist agent, as a cross-protective vaccine is now available and a large proportion of the general population would already have crossreactive antibodies. This vaccine should also serve as an additional layer of safety for researchers working with the 1918 influenza virus. 2009 H1N1 vaccine protects mice from a lethal 1918 virus challenge It was recently found that the 2009 H1N1 pandemic virus shows antigenic similarities to 1918-like and classical swine H1N1 viruses [6] , [7] , [8] , [9] . Here, we evaluated whether immunization of mice with the 2009 H1N1-inactivated vaccine would elicit cross-protective antibodies capable of conferring protection against the more lethal 1918 pandemic influenza virus. At 21 days after vaccination, animals that contained haemagglutination inhibition (HI) titres of ≥40 against homologous virus were selected and matched for challenge experiments. C57B/6 mice immunized with an inactivated 6:2 vaccine engineered with the six internal genes of A/Puerto Rico/8/34 and that contained the HA and neuraminidase (NA) genes of the pandemic H1N1 A/California/04/2009 (Cal/09) strain that had post-vaccination HI titres of 160–1280 were protected from death and exhibited limited morbidity (reduced weight loss) after a 1918 virus lethal challenge with 300 times the 50% lethal dose (300 LD 50 ; 7.35×10 4 plaque-forming units (p.f.u. ); Fig. 1a,b ). This protection was similar to that observed in mice vaccinated with homologous virus-like particles (VLPs) containing the 1918 HA (A/South Carolina/1/18) and NA (A/Brevig Mission/1/18) that exhibited post-vaccination HI titres of 40–640, and contrasted sharply with the level of morbidity and/or mortality observed when a contemporary seasonal H1N1 (A/Brisbane/59/2007 (Bris/59/07))- or H3N2 (A/Brisbane/10/2007 (Bris/10/07))-inactivated vaccine was administered (both eliciting post-vaccination HI titres of 80–640 and 40–160, respectively; Fig. 1a,b ). This difference in morbidity between the Cal/09 and Bris/59/07 vaccine groups was not due to slight differences in HI titres, as, when animals containing the same level of neutralizing antibodies from both groups were compared individually, the magnitude of the weight loss was consistently higher in Bris/59/07 immunized mice ( Fig. 1a ). In addition, Cal/09- and 1918-vaccinated animals had lower virus titres in their lungs compared with seasonal vaccine controls ( Fig. 1c ), indicating an equivalent protective efficacy of the Cal/09 vaccine in mice. 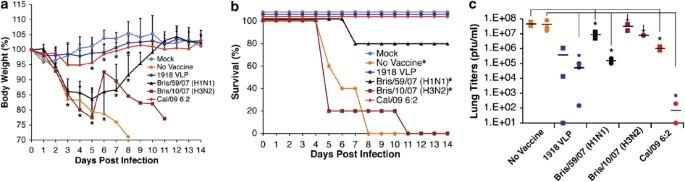Figure 1: An inactivated 2009 H1N1 vaccine elicits cross-protective antibodies against the 1918 pandemic H1N1 virus in mice. (a–c)C57B/6mice (5 weeks old) were immunized twice intramuscularly (at 28 and 14 days before lethal challenge with 300 LD50of 1918 influenza virus on day 0) with 15 μg of the indicated inactivated virus or with 1918 VLP. The mock-infected group received PBS instead of virus challenge. Mice were 9 weeks old at the time of challenge. (a) Body weights represent the average ofn=5 mice per immunization strategy and error bars represent s.d. of mice remaining at each time point. Asterisks below data points represent statistical significant differences in weights, determined by an unpaired Student'st-test (P<0.05), for the no vaccine, Bris/59/07 (H1N1) and Bris/10/07 (H3N2) vaccination groups for days 3–8 (when more than three mice were remaining in each group); and for Cal/04 at the indicated time points, as compared with the mock group. (b) Percentage survival was calculated from the groups above (n=5 mice per group). The log-rank test was used to determine significance (*P<0.05). (c) Viral titres in lungs of vaccinated mice on days 2 (squares) and 4 (circles) after challenge. Titres are shown for two (black arrows) or three mice per group at each time point. Black bars represent the average values, and statistical significance using an unpaired two-tailed Student'st-test (*P<0.05) was determined as compared with the 'no vaccine' control groups. Figure 1: An inactivated 2009 H1N1 vaccine elicits cross-protective antibodies against the 1918 pandemic H1N1 virus in mice. ( a–c ) C57B/6 mice (5 weeks old) were immunized twice intramuscularly (at 28 and 14 days before lethal challenge with 300 LD 50 of 1918 influenza virus on day 0) with 15 μg of the indicated inactivated virus or with 1918 VLP. The mock-infected group received PBS instead of virus challenge. Mice were 9 weeks old at the time of challenge. ( a ) Body weights represent the average of n =5 mice per immunization strategy and error bars represent s.d. of mice remaining at each time point. Asterisks below data points represent statistical significant differences in weights, determined by an unpaired Student's t -test ( P <0.05), for the no vaccine, Bris/59/07 (H1N1) and Bris/10/07 (H3N2) vaccination groups for days 3–8 (when more than three mice were remaining in each group); and for Cal/04 at the indicated time points, as compared with the mock group. ( b ) Percentage survival was calculated from the groups above ( n =5 mice per group). The log-rank test was used to determine significance (* P <0.05). ( c ) Viral titres in lungs of vaccinated mice on days 2 (squares) and 4 (circles) after challenge. Titres are shown for two (black arrows) or three mice per group at each time point. Black bars represent the average values, and statistical significance using an unpaired two-tailed Student's t -test (* P <0.05) was determined as compared with the 'no vaccine' control groups. Full size image 2009 H1N1 human-positive sera protect against the 1918 virus We next evaluated whether vaccination with a 2009 H1N1 licensed inactivated vaccine, used in the 2009/2010 Northern Hemisphere winter season, elicited 1918 crossreactive antibodies in humans. We found that volunteers, 19–82 years of age, who mounted a medium to robust antibody response after a single dose of 2009 H1N1 vaccine (HI titres of ≥40), also displayed significant 1918 influenza HI titres (≥20, Table 1 ). This response is specific, as volunteers that received only seasonal trivalent inactivated vaccine containing H1N1 (Bris/59), H3N2 (Bris/10) and influenza B (B/Brisbane/60/2008) viruses did not have >40 HI titres against Cal/09 or 1918 ( Table 1 ). We tested whether these positive polyclonal human antibodies were capable of protecting mice against a lethal 1918 virus challenge. 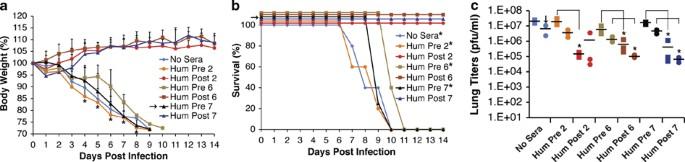Figure 2: Passive immunization with post-vaccination 2009 H1N1 human-positive sera protects mice from 1918 virus lethality. (a–c) 9-week-old mice were treated with a single dose of 100 μl of the indicated human sera or PBS (no sera) intraperitoneally 24 h before challenge with 50 LD50of 1918 virus. (a) Average body weights ofn=4–5 mice per group (black arrow denotes group with four animals), with error bars representing the s.d. for mice remaining at each time. Time points in which the body weight of all the human pre-vaccination groups is significantly different from their respective human post-vaccination group are shown (*P<0.05), as determined by an unpaired two-tailed Student'st-test. (b) Survival curves are shown for the mice groups in (a). The log-rank test was used to evaluate significance (*P<0.05) for survival outcome, black arrow indicates group with four animals. (c) Lung viral titres in passively immunized mice on days 2 (squares) and 4 (circles) after challenge. Viral titres of two (shown with black arrow) or three mice per group per time point are shown as inFigure 1. Significantly different data points (*P<0.05) between the corresponding pre- and post-sera immunizations are shown for each group, as determined by an unpaired two-tailed Student'st-test. Mice passively immunized with undiluted human post-vaccination sera (100 μl) had HI titres of 20–80 against the 1918 virus ( Table 2 ) at the time of infection and were fully protected from a 50 LD 50 (1.19×10 4 p.f.u.) 1918 virus challenge ( Fig. 2a,b ). In contrast, mice administered pre-vaccination sera or that received no treatment as control (no sera) all succumbed to infection by day 10. Furthermore, mice treated with post-vaccination human sera demonstrated a 32- to 141-fold reduction in viral burden in the lungs as compared with controls on day 2 ( Fig. 2c ). At day 4 after challenge, some mice showed an increased viral titre in the lungs as compared with day 2, possibly because of waning antibody levels. However, these mice did not exhibit overt signs of disease, as evidenced by weight loss, lethargy and difficulty in breathing or mortality. In addition, we evaluated whether neutralizing mAbs raised against Cal/09 HA, which map to antigenic site Sa [6] (see Methods), were sufficient to protect mice against a lethal challenge with the 1918 virus. Administration of two neutralizing mouse anti-Cal/09 HA mAbs protected mice from morbidity and mortality against lethal challenge at levels equivalent to administration of a neutralizing mAb raised against the 1918 HA ( Fig. 3a,b ). Virus was undetectable in the mice passively immunized with either 1918- or Cal/09-neutralizing mAbs at both time points analysed ( Fig. 3c ). Overall, these data indicate that the 2009 H1N1 licensed vaccine elicits neutralizing antibodies sufficient to confer full cross-protection to a lethal 1918 pandemic influenza virus challenge. Table 1 HI titres of pre- and post-vaccination human sera against Cal/09 (homologous) and 1918 (heterologous) HA. Full size table Table 2 Cal/09 and 1918 HI titres of mice sera 24 h after passive immunization with pre- and post-vaccination human sera. Full size table Figure 2: Passive immunization with post-vaccination 2009 H1N1 human-positive sera protects mice from 1918 virus lethality. ( a–c ) 9-week-old mice were treated with a single dose of 100 μl of the indicated human sera or PBS (no sera) intraperitoneally 24 h before challenge with 50 LD 50 of 1918 virus. ( a ) Average body weights of n =4–5 mice per group (black arrow denotes group with four animals), with error bars representing the s.d. for mice remaining at each time. Time points in which the body weight of all the human pre-vaccination groups is significantly different from their respective human post-vaccination group are shown (* P <0.05), as determined by an unpaired two-tailed Student's t -test. ( b ) Survival curves are shown for the mice groups in ( a ). The log-rank test was used to evaluate significance (* P <0.05) for survival outcome, black arrow indicates group with four animals. ( c ) Lung viral titres in passively immunized mice on days 2 (squares) and 4 (circles) after challenge. Viral titres of two (shown with black arrow) or three mice per group per time point are shown as in Figure 1 . Significantly different data points (* P <0.05) between the corresponding pre- and post-sera immunizations are shown for each group, as determined by an unpaired two-tailed Student's t -test. 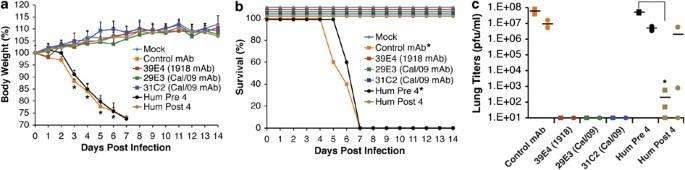Figure 3: Passive immunization with Cal/09-HA specific antibodies and 2009 H1N1 human-positive sera protects mice from 1918 virus lethality. (a–c) mice (9 weeks old) were treated with a single dose of either 150 μg of each mAb (150 μl final volume) or 100 μl of human sera intraperitoneally 24 h before challenge with 50 LD50of 1918 virus, or mock challenged with PBS (mock group). (a) Body weights represent the average fromn=5 mice per immunization strategy and error bars represent s.d. of mice remaining at each time point. Statistical significance (*P<0.05) was determined by an unpaired two-tailed Student'st-test for the control mAb group as compared with the mAb treatment groups, and for the human pre-sera as compared with the human post-sera treatment group. (b) Percentage survival ofn=5 mice per group. Statistical differences (*P<0.05) are shown as compared as above and were determined by the log-rank test. (c) Lung viral titres of passively immunized mice on days 2 (squares) and 4 (circles) after challenge. Viral titres forn=3 mice per group per time point are shown with their respective average represented as black bars. Significant differences (*P<0.05) in viral titres were determined by an unpaired two-tailed Student'st-test. Full size image Figure 3: Passive immunization with Cal/09-HA specific antibodies and 2009 H1N1 human-positive sera protects mice from 1918 virus lethality. ( a–c ) mice (9 weeks old) were treated with a single dose of either 150 μg of each mAb (150 μl final volume) or 100 μl of human sera intraperitoneally 24 h before challenge with 50 LD 50 of 1918 virus, or mock challenged with PBS (mock group). ( a ) Body weights represent the average from n =5 mice per immunization strategy and error bars represent s.d. of mice remaining at each time point. Statistical significance (* P <0.05) was determined by an unpaired two-tailed Student's t -test for the control mAb group as compared with the mAb treatment groups, and for the human pre-sera as compared with the human post-sera treatment group. ( b ) Percentage survival of n =5 mice per group. Statistical differences (* P <0.05) are shown as compared as above and were determined by the log-rank test. ( c ) Lung viral titres of passively immunized mice on days 2 (squares) and 4 (circles) after challenge. Viral titres for n =3 mice per group per time point are shown with their respective average represented as black bars. Significant differences (* P <0.05) in viral titres were determined by an unpaired two-tailed Student's t -test. Full size image Initial concerns about the safety of working with the highly pathogenic 1918 virus called for the development of a vaccine [10] . The data presented in this study indicate that immunization of humans with the 2009 H1N1-inactivated vaccine or natural infection with the 2009 H1N1 virus will confer protective antibody responses against the 1918 pandemic influenza virus in the general population. In addition, although substantial morbidity (body weight loss) was observed in mice immunized with the seasonal H1N1 (Bris/59), this vaccine offered partial protection from death after a 1918 lethal challenge, a phenomenon that has been previously described for heterologous (antigenically different) H1N1 virus strains [6] , [11] . The underlying mechanism responsible for this partial protection is unclear and is thought to be mainly due to anti-HA immune responses [11] , although the activity of antibodies against other viral proteins cannot be ruled out. Nevertheless, this partial cross-protection provides additional indirect evidence that humans vaccinated against or exposed to previous seasonal H1N1 strains might have variable levels of cross-protective immunity against the 1918 virus. Our studies with mAbs further demonstrate that site Sa is an important cross-protective epitope, and thus provide a mechanistic explanation to the high level of cross-protection seen in this study and previously among the 1918 and the Cal/09 vaccines [6] . Our results obtained with the mouse model pave the way for further evaluation of the efficacy of the 2009 H1N1 pandemic vaccine strain in its ability to protect against 1918 virus. Thus, it will be valuable to establish the level of protection that this vaccine would elicit in other animal models, particularly in guinea-pigs, ferrets and monkeys, which will be helpful in assessing morbidity, shedding and in establishing whether vaccination can prevent contact and/or aerosol transmission of the virus. It is important to note that the spread of the 2009 H1N1 influenza virus in the population worldwide, in addition to the large number of individuals already vaccinated, suggests that a large proportion of the population now have cross-protective antibodies against the 1918 virus, considerably reducing the concerns of the consequences of an unwanted or malicious release of this lethal strain of influenza virus. In addition, the wide availability of the 2009 H1N1 virus vaccine should greatly alleviate some of the biosafety and biosecurity concerns voiced at the time of the reconstruction of the 1918 virus. Moreover, our data will likely affect the development of future biosafety measures and policies for working with the 1918 influenza A virus, as immunization with the current 2009 H1N1 vaccine should provide an additional layer of safety for scientists conducting research with this virus. Cell lines and virus strains Human embryonic kidney (293T) cells were maintained in Dulbecco's modified Eagle's medium supplemented with 10% fetal bovine serum (FBS) and 1000 U ml −1 of penicillin/streptomycin. Madin–Darby canine kidney (MDCK) cells were maintained in minimum essential medium supplemented with 10% FBS and penicillin/streptomycin. Cell culture reagents were from Gibco Life Technologies. The H1N1 viruses used in this study are as follows: the recombinant 1918 virus (1918) bearing the HA from A/South Carolina/1/18 and the other seven genes from A/Brevig Mission/1/18, A/Puerto Rico/8/34-MSSM (PR8), Bris/59/07 and Cal/09. The Bris/10/07 virus strain was used as an H3N2 control. Experiments involving 2009 H1N1 and 1918 pandemic viruses were conducted under Biosafety level 3-enhanced conditions in accordance with guidelines of the United States Centers for Disease Control and Prevention. The 1918 virus stocks were grown in MDCK cells. All other viruses were grown in 10-day-old eggs at 37°C for 2–3 days. Vaccine preparation We generated a recombinant influenza A virus carrying HA/NA from Cal/09 and the internal six genes from PR8 (referred to as Cal/09 6:2 in the reminder of the paper) [12] , by transfecting 293T cells with eight ambisense pDZ vectors encoding the eight viral genes and proteins. At 24 h after transfection, the supernatant was collected and inoculated into 8-day-old embryonated chicken eggs. After 3 days of incubation at 35°C, the allantoic fluid containing the rescued virus was plaque purified in MDCK cells. For virus vaccines, viruses were grown once in 10-day-old embryonated chicken eggs at 37°C for 2 days [6] . The allantoic fluid was clarified by low-speed centrifugation at 2,000 g for 10 min at 4°C. Viruses were pelleted on a 30% sucrose cushion by centrifugation at 85,000 g in a SW28 rotor (Beckman Coulter) for 2 h at 4°C. Viral pellets were resuspended in calcium borate buffer pH=7.0 (143 mM sodium chloride, 10 mM calcium chloride, 20 mM boric acid and 2.5 mM sodium borate) at a concentration of 1 mg ml −1 . The viruses were inactivated by formaldehyde (0.9% final concentration). The 1918 virus-based vaccine consisted of VLPs obtained by co-transfection of HA (A/South Carolina/1/18) and NA (A/Brevig Mission/1/18) into 293T cells [13] . The released VLPs were collected and purified from the culture supernatant on a 30% sucrose cushion by centrifugation for 2 h at 85,000 g in an SW28 rotor. Immunization doses were based on the amount of total protein concentration measured by the Bradford method, and seroconversion was assessed on day 21 after vaccination. Site Sa HA-specific mouse mAbs The HA-specific mouse mAbs 29E3 and 39E4 against the pandemic H1N1 2009 and 1918 viruses, respectively, are described in Manicassamy et al [6] . The mAb 31C2 against 2009 H1N1 HA was generated by the hybridoma shared research facility at Mount Sinai School of Medicine, New York. We infected 6-week-old BALB/C mice intranasally with 5×10 4 p.f.u. of influenza virus Cal/09. To boost Cal/09 HA-specific B cells, mice were given an intravenous dose (2×10 7 p.f.u.) of Cal/09 6:2 virus 4 weeks later. On day 3 after the boost, spleens were collected and B cells were fused with SP2/0 myeloma cells by addition of polyethylene glycol. Supernatants from the resulting hybridomas were screened by immunofluorescence staining of 293T cells transfected with the HA expression plasmid, pDZ-HA (Cal/09). Positive hybridomas were subcloned and re-screened. The antibody was isotyped as IgG2b using the IsoStrip kit (Roche) and purified using a Protein A sepharose column. Cal/09 escape mutant viruses containing a G172E mutation (H3 numbering=G158E) in the HA protein were generated by incubating Cal/09 virus with excess 31C2 antibody for 1 h at room temperature (RT). The mixture was inoculated into 10-day-old embryonated eggs and incubated at 37°C for 48 h. Viruses that displayed loss of HI activity against this mAb were amplified and sequenced directly from the reverse transcription–PCR product. Ethics statement and human specimens All research studies involving the use of human specimens were reviewed and approved by the Institutional Review Boards of Saint Louis University School of Medicine and of Mount Sinai School of Medicine. Pre- and post-vaccination human sera samples were obtained from subjects who were 18 years of age or older, who were enrolled in clinical trials to test the safety and immunogenicity of an inactivated 2009 H1N1 influenza vaccine at the National Institute of Allergy and Infectious Disease Vaccine and Treatment Evaluation Unit at Saint Louis University. Experiments to test the reactivity of these sera against the 1918 and Cal/09 HAs were conducted blind. HI assay Mouse and human sera were inactivated using a trypsin-heat-periodate treatment [6] , [14] . We mixed one volume of sera with half a volume of trypsin 8 mg ml −1 (Sigma-Aldrich) in 0.1 M phosphate buffer, pH 8.2, and incubated the samples for 30 min at 56°C. The samples were cooled to RT, mixed with three volumes of 0.11 M metapotassium periodate and incubated for 15 min at RT. The samples were then mixed with three volumes of 1% glycerol saline and further incubated for 15 min at RT. A final 2.5 volumes of 85% saline were added to dilute the samples to a concentration of 1:10. HI assays of mAbs and sera were conducted following standard protocols [13] . Briefly, two-fold serial dilutions of mouse, human sera or mAbs were mixed and pre-incubated in 96-well plates for 30 min at 4°C with 8 HA units of virus per well. Turkey red blood cells were added at a final concentration of 0.25%, and the plate was incubated at 4°C for 30 min. HI titres were determined as the highest dilution that displayed haemagglutinating activity. Specific HI activity of mAbs was calculated as the lowest concentration of mAb that displayed haemagglutinating activity. Mouse experiments C57BL/6 female mice (Jackson Laboratories) were anaesthetized with ketamine–xylaxine intraperitoneally and intranasally infected with the indicated dose of virus diluted in 50 μl of PBS. All animal procedures performed in this study are in accordance with Institutional Animal Care and Use Committee (IACUC) guidelines, and have been approved by the IACUC of Mount Sinai School of Medicine. Mice showing ≥25% of body weight loss were considered to have reached the experimental end point and were humanely euthanized. To obtain viral lung titres, lungs of infected mice were excised on days 2 and 4 after infection and homogenized using a mechanical homogenizer (MP Biochemicals). Virus in homogenates was quantified by plaque assay on MDCK cells. For immunization studies, 5-week-old female C57BL/6 mice were administered 15 μg of inactivated virus or 1918 VLP by intramuscular injection in the hind leg. Two weeks later, a second dose of the same amount of inactivated virus was given as a boost. Four weeks after initial vaccination, the mice were challenged with 300 LD 50 of the 1918 virus. For passive immunizations, 9-week-old C57BL/6 female mice were administered (intraperitoneally) 100 μl of undiluted pre- and post-vaccination human sera, from volunteers immunized with the pandemic 2009 H1N1-inactivated vaccine ( Table 1 ) or 150 μg of the indicated mAb, 24 h before lethal challenge with 50 LD 50 of the 1918 virus. Survival and body weight loss were monitored for 14 days after challenge, and lung viral titres were obtained on days 2 and 4 after challenge. All mice were 9–10 weeks old at the time of lethal challenge. Statistical analysis Statistical significance ( P <0.05) was determined using a two-tailed unpaired Student's t -test for body weight changes and lung viral titres as described in each figure. A log-rank test was used to establish significant differences ( P <0.05) for survival curves. How to cite this article: Medina, R. A. et al . Pandemic 2009 H1N1 vaccine protects against 1918 Spanish influenza virus. Nat. Commun. 1:28 doi: 10.1038/ncomms1026 (2010).